Functional genomics identifies type I interferon pathway as central for host defense againstCandida albicans Candida albicans is the most common human fungal pathogen causing mucosal and systemic infections. However, human antifungal immunity remains poorly defined. Here by integrating transcriptional analysis and functional genomics, we identified Candida -specific host defence mechanisms in humans. Candida induced significant expression of genes from the type I interferon pathway in human peripheral blood mononuclear cells. This unexpectedly prominent role of type I interferon pathway in anti- Candida host defence was supported by additional evidence. Polymorphisms in type I interferon genes modulated Candida -induced cytokine production and were correlated with susceptibility to systemic candidiasis. In in vitro experiments, type I interferons skewed Candida -induced inflammation from a Th17 response towards a Th1 response. Patients with chronic mucocutaneous candidiasis displayed defective expression of genes in the type I interferon pathway. These findings indicate that the type I interferon pathway is a main signature of Candida -induced inflammation and has a crucial role in anti- Candida host defence in humans. C andida albicans is a commensal microorganism that inhabits human skin and mucosa. Candida can be isolated from up to 70% of the general population at any given moment, and it is believed that all individuals have been colonized with Candida at a some point [1] . Although it is a commensal organism, C. albicans can also cause mucosal and systemic infections, especially in immunocompromised hosts [2] . Despite the availability of novel classes of antifungal agents (for example, azoles, echinocandins), mortality due to systemic candidiasis, the fourth most common form of sepsis [3] , [4] , [5] , reaches 37–44% (refs 3 , 6 , 7 ). In addition, vaginal and oral candidiasis can also occur in healthy or only mildly immunocompromised individuals [8] , with up to 5% of women in the general population suffering from recurrent vulvovaginal candidiasis [9] . Despite the introduction of modern antifungal drugs and intensive care facilities, progress in improving the outcome of Candida infections in the last decade has been disappointing. Given this lack of progress, it is currently believed that only adjuvant immunotherapy will be able to further reduce the burden of morbidity and mortality caused by C. albicans infections [10] . Understanding the host defence pathways involved in candidiasis is therefore crucial for identifying novel targets for immunotherapy. To date, all investigations aimed at identifying antifungal host defence mechanisms in humans have relied on candidate-target approaches that are based on biologic plausibility of hypotheses extracted from in vitro or animal studies. Although this approach has been fruitful in confirming important pathways of antifungal defence, it has lacked the power to provide a hierarchy of the importance of these pathways, and to identify potentially novel and unexpected host defence mechanisms against Candida . In the present study, we have taken an alternative, unbiased approach to this biological problem. Using a combination of transcriptional analysis and systems biology, we have stimulated human primary cells with the fungus, identifying Candida -specific transcription profiles in human immune cells. Although C. albicans induced the transcription of multiple inflammatory gene sets commonly stimulated by other inflammatory stimuli, it also specifically induced several additional gene sets, among which we identified an unexpectedly strong type I interferon (IFN) signature profile. We confirmed the importance of the type I IFN pathway for anti- Candida host defence in humans through immunological and genetic studies in both healthy volunteers and in patients with systemic candidiasis or suffering from chronic mucocutaneous candidiasis (CMC). C. albicans induces a type I IFN response We measured genome-wide transcriptional profiles in peripheral blood mononuclear cells (PBMCs) from healthy volunteers upon stimulation with C. albicans , as well as with inflammatory stimuli unrelated to fungal pathogens: Escherichia coli -derived lipopolysaccharide (LPS), Borrelia burgdorferi , Mycobacterium tuberculosis (MTB) and RPMI culture medium as a control. Measurements were performed at 4 and 24 h. A total of 693 transcripts that showed >2-fold higher expression compared with corresponding RPMI stimulation were selected (Benjamini and Hochberg’s (BH)-adjusted P <0.05). K-means analysis identified profile clusters that indicated shared and specific genes that were differentially expressed in response to each stimulus. We grouped shared genes into signatures representing common early response genes (clusters 1, 6, 14, 27), common late response genes (clusters 2, 3) and common inflammatory genes induced by all stimulations (clusters 9, 21, 25) ( Fig. 1a and Supplementary Figs S1–S3 ). 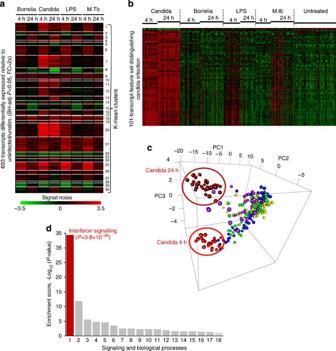Figure 1: Transcriptional responses to Candida. (a) K-means clustering identifies shared and specific gene signatures in response to infection or stimulation. For example, clusters 21 and 25 indicate common inflammatory genes (details inSupplementary Fig. S2) that are significantly differentially induced genes (Benjamini–Hochberg-adjustedP<0.05, fold change>2) in response toB. burgdorferi,C. albicans,E. coli-derived LPS andMycobacterium tuberculosis(M.tb), compared with RPMI stimulations (Untreated), while clusters 7, 11 and 20 identifyCandida-dominant response genes. Signal-to-noise ratio relative to untreated is shown in the heatmap. (b) Using feature selection, naïve Bayes classifier and 10-fold cross-validation, a 101-transcript feature set was identified from 693 differentially expressed transcripts shown ina, which distinguishesCandidafrom the other stimulants and an area under the ROC (receiver-operating characteristic) curve of 97.8%, indicating a high discriminative value. The expression profile (Z-transformed) of this feature set is displayed. (c) Principal component analysis (PCA) of theCandida-response signature. Data from each individual sample is plotted along the three main principal components (PC1, PC2, PC3). The three main principal components account for 45% of the total variance in gene expression. Samples from the various stimulations and infections are colour coded as follows:C. albicans(2 h: bright red; 24 h: dark red),B. burgdorferi(Green),E. coli-derived LPS (Blue), M.tb (Purple) and untreated (Yellow). (d) Enrichment analysis (MetaCore pathways) of the 101-transcript feature set reveals a striking enrichment of the IFN signalling pathway.Supplementary Table S2displays all the signalling/biological processes shown and their enrichmentP-values. Figure 1: Transcriptional responses to Candida. ( a ) K-means clustering identifies shared and specific gene signatures in response to infection or stimulation. For example, clusters 21 and 25 indicate common inflammatory genes (details in Supplementary Fig. S2 ) that are significantly differentially induced genes (Benjamini–Hochberg-adjusted P <0.05, fold change>2) in response to B. burgdorferi , C. albicans , E. coli -derived LPS and Mycobacterium tuberculosis (M.tb), compared with RPMI stimulations (Untreated), while clusters 7, 11 and 20 identify Candida -dominant response genes. Signal-to-noise ratio relative to untreated is shown in the heatmap. ( b ) Using feature selection, naïve Bayes classifier and 10-fold cross-validation, a 101-transcript feature set was identified from 693 differentially expressed transcripts shown in a , which distinguishes Candida from the other stimulants and an area under the ROC (receiver-operating characteristic) curve of 97.8%, indicating a high discriminative value. The expression profile ( Z -transformed) of this feature set is displayed. ( c ) Principal component analysis (PCA) of the Candida -response signature. Data from each individual sample is plotted along the three main principal components (PC1, PC2, PC3). The three main principal components account for 45% of the total variance in gene expression. Samples from the various stimulations and infections are colour coded as follows: C. albicans (2 h: bright red; 24 h: dark red), B. burgdorferi (Green), E. coli -derived LPS (Blue), M.tb (Purple) and untreated (Yellow). ( d ) Enrichment analysis (MetaCore pathways) of the 101-transcript feature set reveals a striking enrichment of the IFN signalling pathway. Supplementary Table S2 displays all the signalling/biological processes shown and their enrichment P -values. Full size image More importantly, to identify a set of discriminatory features (from the 693 differentially expressed transcripts) that would be most informative of the state of Candida stimulation and could distinguish Candida stimulation from the other inflammatory stimuli, we utilized information gain (Kullback–Leibler divergence/relative entropy) feature selection, to reduce the dimensionality of the feature space [11] , [12] . We performed 10-fold cross-validation that stratifies the data into 10 random partitions in which each (in turn) is held out for testing and the remainder for training a Bayesian classifier. Class prediction was evaluated by computing the area under the receiver-operating characteristic curve, which assesses true- and false-positive rates. A 101-transcript (95-gene) Candida -response signature ( Fig. 1b and Supplementary Table S1 ) was defined using this supervised learning approach for class prediction, achieving an area under the receiver-operating characteristic curve of 97.8%, which would indicate an excellent classifier performance with very high discriminative value. Principal component analysis of the Candida -response signature further demonstrated good class separation on the basis of Candida status and stimulation duration ( Fig. 1c ). As a set, the 101 features collectively identify expression signatures that are informative of Candida stimulation across the 4, 24-h or both time points that sufficiently distinguish Candida from the rest. Enrichment analysis for the 101 transcript Candida -response signature revealed a striking overrepresentation of the IFN signalling pathway ( P =3.8 × 10 −35 ) ( Fig. 1d and Supplementary Table S2 ). This set of genes was strongly induced at both 4 and 24 h of Candida stimulation and establishes a definitive Candida -responsive signature distinct from that observed with LPS, MTB or Borrelia stimulation. Type I IFN SNPs modulate susceptibility to candidemia To assess whether the type I IFN genes specifically induced by C. albicans in human leukocytes are indeed involved in antifungal host defence, we investigated whether common polymorphisms in a subset of these genes influence susceptibility to systemic Candida infections. From a cohort of 217 Caucasian patients with candidemia, well described elsewhere [10] , [13] , we had Immunochip genotyping data available and 11 genes of the 101-transcript (95-gene) data set were covered by the Immunochip array ( Supplementary Table S3 ). We tested these 11 genes for association by taking immunochip data on 12,228 non-candidemia Caucasian healthy volunteers as controls [14] . Analysis of the loci associated with these 11 genes revealed significant association of genetic variation with susceptibility to systemic candidiasis in four regions: CCL8 SNP 1kg_17_29697448 ( P =0.00069), STAT1 SNP rs16833172 ( P =0.0042), SP110 SNP rs3769845 ( P =0.012) and PSMB8 SNP rs3198005 ( P =0.01) ( Fig. 2a–d ; Supplementary Figs S1–S3 , clusters 10, 11, 20, 11, respectively) ( Supplementary Table S3 ). After applying a stringent Bonferroni correction for multiple testing, the association between susceptibility to candidemia and STAT1 and CCL8 remained significant. This finding confirms that the C. albicans -specific genes we identified in our transcriptional arrays have an important role in host defence against systemic fungal infections. We also attempted to assess whether the polymorphisms in these genes also modified disease severity. However, only 51 patients fulfilled the criteria of severe candidiasis based on clinical scores and persistence of positive blood cultures, and this number was too low for allowing the identification of significant differences between genetic variation and disease severity (disseminated disease, persistent fungemia and mortality at 14 or 30 days) (data not shown). 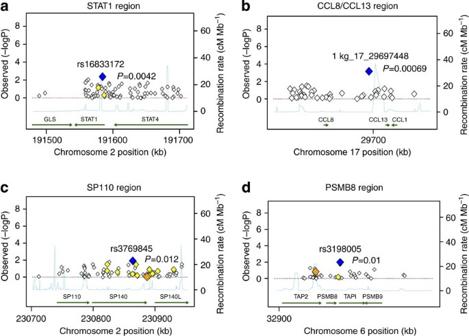Figure 2: SNPs of type I IFN-responsive genes are associated with susceptibility to Candidemia. Regional association plots, at (a)STAT1region (b)CCL8/CCL13region (c)SP110region and (d)PSMB8region, showing chromosome position in thexaxis and the –log of logisticP-values for each SNP in theyaxis. Blue diamond indicates the topP-value; whereas orange and yellow diamonds indicatesr2ranges of 0.6–0.8 and 0.4–0.59, respectively, with the top-associated SNP. SNP names shown are as in dbSNP130 where available. Otherwise, the Illumina Immunochip manifest name is shown. For example, 1kg_17_29697448 indicates the location of SNP on chromosome 17 at position 29697448 (hg18). Figure 2: SNPs of type I IFN-responsive genes are associated with susceptibility to Candidemia. Regional association plots, at ( a ) STAT1 region ( b ) CCL8/CCL13 region ( c ) SP110 region and ( d ) PSMB8 region, showing chromosome position in the x axis and the –log of logistic P -values for each SNP in the y axis. Blue diamond indicates the top P -value; whereas orange and yellow diamonds indicates r 2 ranges of 0.6–0.8 and 0.4–0.59, respectively, with the top-associated SNP. SNP names shown are as in dbSNP130 where available. Otherwise, the Illumina Immunochip manifest name is shown. For example, 1kg_17_29697448 indicates the location of SNP on chromosome 17 at position 29697448 (hg18). Full size image Type I IFN SNPs modulate Candida -induced cytokine responses In an additional approach to validate the role of the type I IFN pathway for host defence against Candida , we isolated PBMCs from an additional group of 74 healthy volunteers and stimulated the cells with the fungus. Genetic variation in 11 type I IFN pathway genes present on the Immunochip was correlated with C. albicans -induced release of tumour-necrosis factor-α (TNF-α), interleukin (IL)-1β, IL-8, IL-6, IL-10, IFN-γ and IL-17. In contrast to other microbial stimuli such as LPS and MTB, C. albicans induced higher levels of TNF-α, IL-1β and IL-10 production, and lower levels of IL-8 and IL-6 in human PBMCs ( Supplementary Fig. S4 ). The correlation of cytokine concentrations with genotypes at tag single nucleotide polymorphisms (SNPs) of Candida -induced IFN pathway genes revealed significant associations at IRF1 and STAT1 regions ( Fig. 3a–d ) in which IRF1 SNPs were associated with TNF-α ( P =0.0028) and IL-10 levels ( P =0.0024), whereas STAT1 SNPs were associated with TNF-α ( P =0.001) and IL-6 levels ( P =0.0002). Consistent with the specificity of the type I IFN pathway for Candida stimulation, the association was significant with cytokine levels induced by Candida , but not by LPS or MTB stimulation ( Supplementary Fig. S5 ). 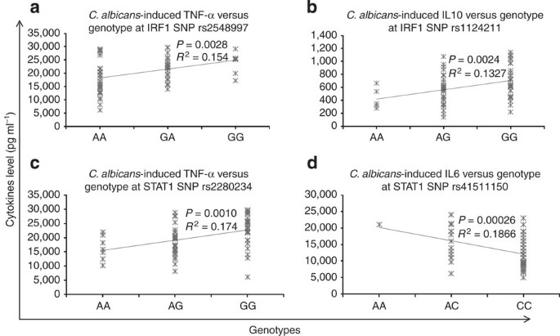Figure 3: SNPs of type I IFN-responsive genes are associated withCandida-induced cytokine levels. Correlation plots showing the association between genotypes in thexaxis and cytokines levels in theyaxis. Association between (a) TNF-α levels and genotypes atIRF1SNP rs2548997, (b) IL-10 levels and genotypes atIRF1SNP rs1124211, (c) TNF-α and genotype atSTAT1SNP rs2280234 and (d) IL-6 levels and genotypes atSTAT1SNP rs41511150. Figure 3: SNPs of type I IFN-responsive genes are associated with Candida -induced cytokine levels. Correlation plots showing the association between genotypes in the x axis and cytokines levels in the y axis. Association between ( a ) TNF-α levels and genotypes at IRF1 SNP rs2548997, ( b ) IL-10 levels and genotypes at IRF1 SNP rs1124211, ( c ) TNF-α and genotype at STAT1 SNP rs2280234 and ( d ) IL-6 levels and genotypes at STAT1 SNP rs41511150. Full size image Type I IFNs skew cytokine responses from Th17 towards Th1 To investigate the importance of type I IFN signalling in host defence against Candida , PBMCs from healthy individuals were stimulated with heat-killed C. albicans . In line with the transcriptional profile described above ( Fig. 1 ), IFN-β could be detected in cell culture supernatants only after C. albicans stimulation. In contrast, neither live ( Fig. 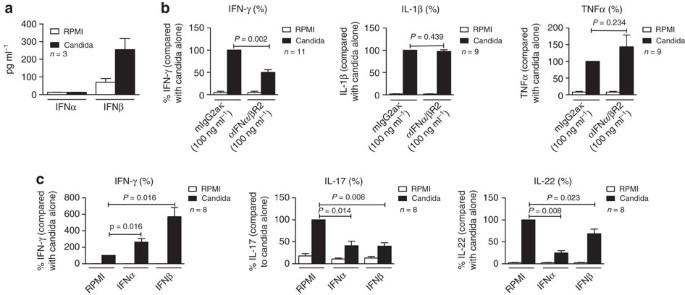Figure 4: Type I IFNs skew cytokine production from a Th1 towards a Th17 response. (a) 5 × 105PBMC in a volume of 200 μl, were stimulated for 7 days, in the presence of 10% human pooled serum, with liveC. albicans(1 × 106ml−1),in duplo. IFN-α and IFN-β were measured in cell culture supernatants using enzyme-linked immunosorbent assay (ELISA). (b) 5 × 105PBMC in a volume of 200 μl, were stimulated for 1 and 2 days, with heat-killedC. albicans(1 × 106ml−1), in the absence or presence of anti-IFN-α/βR2,in duplo. IFN-γ, IL-1β and TNF-α were measured in cell culture supernatants using ELISA. (c) A total of 5 × 105PBMC in a volume of 200 μl, were stimulated for 2 and 7 days, with heat-killedC. albicans(1 × 106ml−1), in the absence or presence of IFN-α or IFN-β,in duplo. When cells were cultured for 7 days, this was done in the presence of 10% human-pooled serum. IFN-γ, IL-17 and IL-22 were measured in cell culture supernatants using ELISA. (a–c) After stimulation, supernatants were pooled and stored at−20 °C until further assayed. Data were analysed using the Wilcoxon-signed rank test. Data are presented as mean+s.e.m. 4a ), nor heat-killed C. albicans induced any detectable IFN-α production Figure 4: Type I IFNs skew cytokine production from a Th1 towards a Th17 response. ( a ) 5 × 10 5 PBMC in a volume of 200 μl, were stimulated for 7 days, in the presence of 10% human pooled serum, with live C. albicans (1 × 10 6 ml −1 ), in duplo . IFN-α and IFN-β were measured in cell culture supernatants using enzyme-linked immunosorbent assay (ELISA). ( b ) 5 × 10 5 PBMC in a volume of 200 μl, were stimulated for 1 and 2 days, with heat-killed C. albicans (1 × 10 6 ml −1 ), in the absence or presence of anti-IFN-α/βR2, in duplo . IFN-γ, IL-1β and TNF-α were measured in cell culture supernatants using ELISA. ( c ) A total of 5 × 10 5 PBMC in a volume of 200 μl, were stimulated for 2 and 7 days, with heat-killed C. albicans (1 × 10 6 ml −1 ), in the absence or presence of IFN-α or IFN-β, in duplo . When cells were cultured for 7 days, this was done in the presence of 10% human-pooled serum. IFN-γ, IL-17 and IL-22 were measured in cell culture supernatants using ELISA. ( a – c ) After stimulation, supernatants were pooled and stored at−20 °C until further assayed. Data were analysed using the Wilcoxon-signed rank test. Data are presented as mean+s.e.m. Full size image We next assessed the role of type I IFN pathways in the induction of cytokines by C. albicans . When PBMCs were stimulated with heat-killed C. albicans in the presence of an antibody against IFN-α/β/ω receptor 1 (IFNAR), IFNγ production was significantly lower compared with PBMCs stimulated in the presence of a control antibody. Blocking of IFNAR did not influence the production of the monocyte-derived cytokines IL-β or TNF-α ( Fig. 4b ). Conversely, adding IFN-α or IFN-β to Candida -stimulated cells increased IFN-γ production, while significantly decreasing IL-17 and IL-22 production ( Fig. 4c ). Together these data indicate that type I IFNs (in the context of infection, most likely IFN-β) modulate the immune reaction induced by C. albicans , skewing host defence towards a Th1 response. STAT1 mutations cause reduced expression of type I IFN genes Patients with autosomal-dominant CMC have increased susceptibility to mucosal fungal infections and often carry gain-of-function mutations in STAT1 (refs 15 , 16 ), which lead to STAT1 hyperphosphorylation, that in turn likely makes STAT1 unavailable for forming heterodimers with other STAT molecules [17] . In co-cultures of dendritic cells (DCs) and T cells from CMC patients, this led to defective Th1 and Th17 responses ( Supplementary Fig. S6 ). To validate the role of Candida -specific genes in human antifungal mucosal defence, we assessed the expression of these genes in cells from CMC patients. PBMCs from healthy controls and CMC patients were stimulated with RPMI, E. coli -derived LPS, heat-killed C. albicans , or heat-killed MTB. The expression of type I IFN pathway genes (including IRF5, IRF7 , ISG15 , IFI44 and IFI44L ) that are induced downstream of STAT1-STAT2 showed patterns of defective expression in CMC patients compared with healthy controls, supporting a role of the type I IFN pathway in this immunodeficiency ( Fig. 5 ). The expression of IRF3, IRF9 and IFN-β , three genes in the type I IFN pathway upstream of STAT1-STAT2, was not decreased in cells from CMC patients. In fact, Candida -induced IFN-β expression appeared to be higher in cells from CMC patients, possibly indicating a compensatory feedback mechanism. 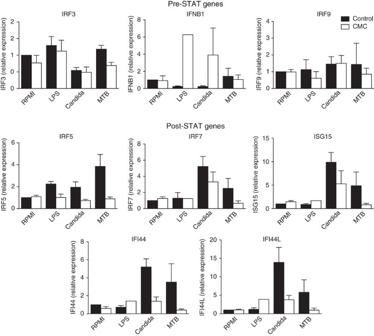Figure 5: Expression of type I IFN pathway genes in patients with a STAT1 mutation. Reduced expression of type I IFN pathway genes in patients with a STAT1 mutation (n=2, with patients measured twice), and healthy controls (n=8). A total of 5 × 105PBMC in a volume of 200 μl, were stimulated for 24 h, with RPMI,E. coli-derived LPS (10 ng ml−1), heat-killedC. albicans(1 × 106ml−1), or heat-killed MTB (1 μg ml−1). mRNA was isolated from cell lysates using TRIzol. Transcription of IFN-β, IRF3, IRF9, IRF5, IRF7, ISG15, IFI44 and IFI44L was measured using quantitative PCR. Data are presented as mean+s.e.m. Figure 5: Expression of type I IFN pathway genes in patients with a STAT1 mutation. Reduced expression of type I IFN pathway genes in patients with a STAT1 mutation ( n =2, with patients measured twice), and healthy controls ( n =8). A total of 5 × 10 5 PBMC in a volume of 200 μl, were stimulated for 24 h, with RPMI, E. coli -derived LPS (10 ng ml −1 ), heat-killed C. albicans (1 × 10 6 ml −1 ), or heat-killed MTB (1 μg ml −1 ). mRNA was isolated from cell lysates using TRIzol. Transcription of IFN-β, IRF3, IRF9, IRF5, IRF7, ISG15, IFI44 and IFI44L was measured using quantitative PCR. Data are presented as mean+s.e.m. Full size image To investigate the type I IFN pathway in CMC patients in a more systematic way, we also performed RNA sequencing analysis in PBMCs stimulated with C. albicans from both control volunteers and CMC patients. The differential expression of 91 genes in response to C. albicans stimulation was compared between CMC patients and healthy controls (10 genes from the 101-gene signature characteristic for Candida were not considered: 7 because another isoform was already used for FPKM (Fragments per Kilobase per Million mapped) calculations, and 3 hypothetical proteins without concordant refseq genes). In cells from healthy controls, two genes showed downregulation ( LFNG, RGC32 ), whereas all other genes were upregulated upon stimulation ( Supplementary Fig. S7 ), validating the previous findings based on expression array analysis. To observe differences between patients and controls, the standardized fold change was used to create the respective heatmap ( Fig. 6 ). The patients show a much lower standardized fold change in genes downstream of STAT1, again supporting the role of type 1 IFN pathway in CMC. We found 27 genes, from the set of 91 genes, to be significantly differently regulated upon Candida stimulation in patients compared with controls based on an analysis of variance (ANOVA) analysis ( P -value interaction group and treatment <0.05) ( MX1, OAS3, IFIT2, RTP4, XAF1, OAS2, IFI44, IFIH1, IFIT3, ADAR, PRIC285, FAM46A, SAMD9L, EIF2AK2, PARP12, TRIM22, ZBP1, HERC6, RSAD2, IFNG, OAS1, STAT2, DHX58, IRF7, TNFSF10, ISG15, HERC5 ). To determine the role of these 27 genes we calculated Gene ontology enrichment scores using the Database for Annotation, Visualization and Integrated Discovery. Enriched gene clusters were generated using Functional Annotation Clustering. Gene ontology terms associated with response to type I IFN and viral infections showed significant enrichment ( P =1.09 × 10 −14 ) ( Supplementary Table S4 ). 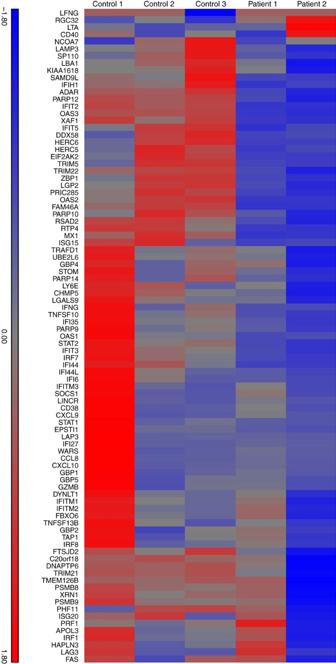Figure 6: Heatmap of response of CMC patients and controls toC. albicans in vitrostimulation. In this analysis the standardized fold change gene expression in stimulated versus unstimulated cells was calculated. The scale of this heatmap is given as standardized log2 fold change with a range from −1.8 (blue) to +1.8 (red). Figure 6: Heatmap of response of CMC patients and controls to C. albicans in vitro stimulation. In this analysis the standardized fold change gene expression in stimulated versus unstimulated cells was calculated. The scale of this heatmap is given as standardized log2 fold change with a range from −1.8 (blue) to +1.8 (red). Full size image The last decade has witnessed a significant increase in knowledge related to the mechanisms involved in antifungal host defence. However, most of this knowledge is based on in vitro and animal studies; these studies led to hypotheses to be tested in human systems, leading to a somewhat biased view of human immunity against fungi. In the present study we have used a different approach based exclusively on complementary human studies: transcriptomics analysis in human primary cells, correlation of genetic variability and antifungal immunity in healthy volunteers (functional genomics), case–control association studies in patients with disseminated C. albicans infections and assessment of antifungal immunity in CMC patients. In our initial approach, we designed a hypotheses-generating set of experiments by assessing the transcriptional profile induced in circulating primary leukocytes by C. albicans . Human primary PBMCs were stimulated either with C. albicans or with other inflammatory stimuli. Pathway analysis of the genes induced by Candida indicated two broad categories: (i) a first set of genes that was strongly induced and shared by both C. albicans and other inflammatory stimuli (LPS, MTB or B. burgdorferi) , constituted expected pathways involved in inflammation and innate immunity, many of which have important roles in antifungal immunity [18] , and (ii) a feature set comprising an expression signature of 101 transcripts (95 genes) that distinguishes the Candida -specific response and is characterized by a strikingly strong and unanticipated type I IFN response. Because the identification of the type I IFN pathway as the most prominent Candida -specific transcriptional signature was surprising, we initiated a series of studies to confirm this finding. First, we assessed whether genetic polymorphisms in several of the genes identified in the Candida -specific data set influenced susceptibility to systemic Candida infections. In a cohort of patients with candidemia that were genotyped using the Immunochip platform (Illumina [14] ), on which 11 genes of the Candida -specific data set were covered, we identified significant association of genetic variation with susceptibility to candidiasis in four of these genes: CCL8 locus, STAT1 , SP110 locus and PSMB8 locus. This finding confirms that genes from the 101 Candida -specific data set influence susceptibility to systemic fungal infections. Second, the role of the type I IFN pathway for the anti- Candida immune response was subsequently validated in a study in which PBMCs isolated from a group of healthy volunteers were stimulated with the fungus. Genetic variation in the 11 type I IFN pathway genes present on the Immunochip was correlated with C. albicans -induced cytokine production. The correlation of cytokine concentrations with genotypes at tag SNPs of Candida -induced IFN pathway genes revealed significant associations at IRF1 and STAT1 regions, both crucial components of type I IFN pathway. We cannot exclude, however, that the effect of these polymorphisms on TNF-α production are exerted through type II IFNs; IFNγ is stimulated by type I IFNs [19] , and is known to induce TNF-α production [20] . These data support the hypothesis of the specificity of the type I IFN pathway for Candida stimulation, as this association was significant only for cytokine production induced by Candida , but not by other stimuli. Third, we performed classical immunological studies to assess the role of type I IFNs for Candida -induced immune responses, and we demonstrated that type I IFNs induced by Candida modulate Th1/Th17 cytokine profiles; IFNα and IFNβ increased IFNγ production, while decreasing IL-17 production. Moschen et al . [21] previously demonstrated that type I IFNs decrease IL-17 production in vitro and in vivo . TNF-α production did not seem to be influenced by blocking the IFNAR, suggesting that genetic effects in STAT1 exert their effect on TNF-α production either through direct intracellular pathways, or indirectly through IFNγ. Interestingly, C. albicans seems to induce only IFN-β, rather than IFN-α, consistent with earlier studies in mice [22] , [23] . Finally, using both quantitative PCR and RNA sequencing analysis, we demonstrated that the expression of type I IFN pathway-induced genes was defective in CMC patients harbouring a gain-of-function mutation in STAT1 (ref.15) [15] . These mutations lead to increased STAT1 phosphorylation and IFNγ signalling. Liu et al . [16] demonstrated increased STAT1 phosphorylation in response to IFNγ stimulation in U3C cells transfected with mutated STAT1. They hypothesize that IFN-targeted genes can lead to decreased IL-17 production. However, freshly isolated PBMC from CMC patients do not produce any IFNγ in response to C. albicans stimulation [15] . Therefore, it is more likely that the inability of mutated STAT1 to form heterodimers with STAT3 and STAT4 causes defective Th1/Th17 responses [17] , which are likely to represent the main immunological defect in this disease. Additional defects in the expression of type I IFN-induced genes, as shown here, may also contribute to the increased susceptibility to mucosal fungal infections. Whether this is truly caused by a defect in STAT1-STAT2 heterodimerization remains to be demonstrated. Taken together, these complementary studies represent a compelling body of evidence that the type I IFN pathway is an important component of the immune response during infections with C. albicans in humans. Moreover, the data presented here are supported by emerging information from murine studies. For example, Bourgeois et al . [22] and Biondo et al . [23] have reported that mouse conventional DCs produce IFN-β upon stimulation with Candida spp. and have proposed a role for MyD88, TLR7 and TLR9 in this induction. On the other hand, these results are relatively surprising, as no earlier study has reported a role for type I IFNs in human antifungal host defence. In this respect, primary immunodeficiencies in type I IFN pathway are mainly associated with viral, rather than fungal, infections [24] . Therefore, our data indicate that type I IFN defects determine an increase susceptibility risk for fungal infections, as demonstrated here by the association with candidemia in risk groups, rather than an overt immunodeficiency associated with severe fungal infections. The precise effect of type I IFNs for anti- Candida host defence is still being debated. One study in type I IFNAR knockout mice suggested a deleterious role for this pathway [22] , whereas another study reported that IFNAR −/− mice die from their inability to control fungal growth [23] . Although type I IFNs have an important role in the immune response against viral infections [25] , they seem to be deleterious in bacterial infections [26] . In humans with Candida infections, the role of type 1 IFNs is not yet settled, although the defects seen in type I IFN gene expression in CMC patients, the susceptibility to candidemia by STAT1 polymorphisms, and the potentiation of Th1 responses by type I IFNs, all suggest a beneficial effect of the type I IFN pathway in human antifungal host defence. Although viruses have long been known to induce type I IFN production, other microorganisms have been recently reported to induce this pathway. MTB stimulation induces the expression of IFNB and IFNA1 in human macrophages [27] and in murine bone marrow-derived macrophages [28] ; type I IFNs are required for caspase-1 activation during Francisella tularensis infection [29] ; and Listeria monocytogenes induces the transcription of IFNB in macrophages [30] . However, the complete transcriptional profile of the type I IFN pathway performed here shows important differences from the type I IFN profile induced by MTB [31] and is significantly more pronounced for Candida than for MTB ( Supplementary Fig. S4 ). Interestingly, the very strong induction of type I IFN pathway genes by Candida may explain the well-known, yet unexplained, beneficial effects of injecting Candida -derived extracts for the treatment of warts in patients [32] , [33] . In summary, this work presents complementary arguments from several studies to propose that the type I IFN pathway has an important role in the immune responses to the fungal pathogen C. albicans in humans. The cross-validation between these approaches supports the value of this systems biology approach, combining transcriptomics with functional genomics and immunological data. Using this approach, we have confirmed the role of pathways known to be involved in antifungal host defence (for example, common inflammatory pathways and the Th1/Th17 pathways) and we have identified a novel pathway (the type I IFN pathway). It is expected that this knowledge will have an important contribution in devising novel immunotherapeutic strategies for fungal infections, as well as influencing decision-making for vaccine design. Study populations For assessing the transcriptome and the cytokine production capacity, blood was collected after written informed consent from healthy volunteers. Adult patients with candidemia were enroled after informed consent (or waiver as approved by the Institutional Review Board) at the Duke University Hospital (DUMC, Durham, North Carolina, USA) and Radboud University Nijmegen Medical Centre (RUNMC, Nijmegen, The Netherlands). The study was approved by the Institutional Review Boards at each study centre, and enrolment occurred between January 2003 and January 2009 (ref. 34 ). The study was performed in accordance with the declaration of Helsinki. In addition, blood was collected from two patients with CMC (on two different occasions) and eight healthy controls to investigate the induction of IFN genes by Candida . After informed consent was given, blood was collected by venipuncture into 10 ml EDTA syringes (Monoject, s-Hertogenbosch, The Netherlands). PBMC isolation Separation and stimulation of PBMCs was performed as described previously [35] . Briefly, the PBMC fraction was obtained by density centrifugation of diluted blood (1 part blood to 1 part pyrogen-free saline) over Ficoll–Paque (Pharmacia Biotech, Uppsala, Sweden). PBMCs were washed twice in saline and suspended in culture medium. The cells were counted in a haemocytometer and their number was adjusted to 5 × 10 6 ml −1 . Cell stimulation For the transcriptome analysis, cells were stimulated for 4 or 24 h with RPMI, heat-killed B. burgdorferi [36] , C. albicans (UC 820) (1 × 10 6 ml −1 ) [37] , MTB (1 μg ml −1 ) or E. coli -derived LPS (10 ng ml −1 ). To correlate cytokine production to SNPs in the type I IFN pathway, 5 × 10 5 PBMCs from healthy volunteers were stimulated with heat-killed C. albicans (1 × 10 6 ml −1 ) for 24 h. To investigate the effect of type I IFNs on cytokine production, 5 × 10 5 PBMCs were stimulated with heat-killed C. albicans (1 × 10 6 ml −1 ) in the absence or presence of IFN-α2b (1 × 10 5 U ml −1 ) (IntronA, SP Labo N.V., Heist-op-den-berg, Belgium), IFN-β (10 ng ml −1 ) or anti-IFNAR (100 ng ml −1 ) (21385-1, PBL Inferon Source, Piscataway, USA). To assess the development of Th1 and Th17 cells, a total of 1 × 10 6 mononuclear cells were added to 96-well flat-bottom plates (Greiner). Subsequently, the monocytes within the PBMC pool were differentiated towards DCs by addition of IL-4 (50 ng ml −1 , R&D Systems), GM-CSF (50 ng ml −1 , R&D Systems) and 10% human serum for 7 days. After every second day, half of the medium was replaced by fresh DC differentiation medium. At day 7 of the culture, cells were stimulated with 1 × 10 6 Candida conidia for another 6 days. Transcriptome analysis Global gene expression was profiled using Illumina Human HT-12 Expression BeadChip according to manufacturer’s instructions. Image analysis, bead-level processing and quantile normalization of array data were performed using the Illumina LIMS platform, BeadStudio. A gene-wise linear model was fitted to the data and was performed in R programming language ( http://www.r-project.org/ ), utilizing functions from Linear Models for Microarray Data [38] . For each probe, a moderated t -statistic (with s.e. moderated across genes) was computed using a Bayesian model. The associated P -values were adjusted to control the false discovery rate in multiple testing, using the BH method [39] . For each transcript, Signal-to-Noise ratios (SNR) were computed for each infection or stimuli group relative to the untreated (RPMI) control group. The expression SNR profiles of transcripts identified as differentially expressed (BH-adjusted P <0.05 and fold-change >2 × ) were clustered using the K-means algorithm [40] . We performed feature (attribute) selection [41] , [42] on differentially expressed transcripts using Information Gain (Kullback–Leibler divergence or relative entropy) to identify discriminatory features or transcripts that are most informative of the state of infection or stimulation. The accuracy of class prediction using a Java implementation of a naïve Bayes classifier [42] , [43] incorporating these features was evaluated using 10-fold cross-validation. Cytokine measurements The concentration of IL-1β, IL-17, IL-22, TNF-α (R&D Systems, Abingdon, UK), IL-6, IL-8, IL-10, IFN-γ (Sanquin, Amsterdam, the Netherlands) and IFN-α, IFN-β (PBL Interferon Source, Piscataway, USA) was measured in cell culture supernatants using enzyme-linked immunosorbent assay according to the instructions of the manufacturer. SNP selection DNA was isolated using the Gentra Pure Gene Blood kit (Quiagen, Venlo, The Netherlands), according to the protocol of the manufacturer. Illumina Immunochip is a custom-designed high-density array to densely genotype 186 loci associated with 12 different autoimmune or inflammatory diseases reaching genome-wide association study significance threshold ( P <5 × 10 −8 ) [14] . The candidemia cohort and volunteers DNA samples were genotyped on this Immunochip Illumina platform. Only SNPs in 11 of the 101-gene data set identified earlier were studied, as the other genes were not represented on the Immunochip. We selected tag-SNPs ( Supplementary Table S3 ) at each region that are located within ±250 kb of the locus by employing Haploview [44] and we excluded SNPs with r 2 ≥0.8 from association analysis. Statistical analysis Analyses were performed using PLINKv1.07 (refs 45 , 46 ). We performed Multidimensional scaling (MDS) analysis to reveal genetic background of cases and controls in Candidemia cohort ( Supplementary Fig. S8 ). The association between tag-SNPs and Candidemia susceptibility was tested by logistic regression with the first four components from MDS analysis as covariates. The correlation between cytokine levels and genotypes was tested by Wilcoxon rank sum test using R. P <0.05 was considered significant. Real-time PCR Two million freshly isolated PBMCs were incubated with various stimuli as described above. After 24 h of incubation at 37 °C, total RNA was extracted in 800 μl of TRIzol reagent (Invitrogen, Breda, The Netherlands). Isolated RNA was reverse-transcribed into complementary DNA using oligo(dT) primers and MMLV reverse transcriptase. PCR was performed using a 7300 Real-Time PCR system (Applied Biosystems, Lennik, Belgium). Primer sequences for human IFN-β: sense: 5′-ATG-ACC-AAC-AAG-TGT-CTC-CTC-C-3′ and antisense: 5′-GGA-ATC-CAA-GCA-AGT-TGT-AGC-TC-3′; IRF9: sense 5′-GAT-ACA-GCT-AAG-ACC-ATG-TTC-CG-3′and antisense: 5′- TGA-TAC-ACC-TTG-TAG-GGC-TCA-3′; IRF7: sense: 5′-GCT-GGA-CGT-GAC-CAT-CAT-GTA-3′ and antisense: 5′-GGG-CCG-TAT-AGG-AAC-GTG-C-3′; ISG15: sense: 5′-CGC-AGA-TCA-CCC-AGA-AGA-TCG-3′ and antisense: 5′-TTC-GTC-GCA-TTT-GTC-CAC-CA-3′; IFI44: sense: 5′-ATG-GCA-GTG-ACA-ACT-CGT-TTG-3′ and antisense: 5′-GCA-GGA-TCT-TTC-GTG-CAA-CC-3′; IFI44L: sense: 5′-AGG-GAA-TCA-TTT-GGC-TCT-GTA-GA-′3 and antisense: 5′-AGC-CGT-CAG-GGA-TGT-ACT-ATA-AC-3′; IRF3: sense: 5′-AGA-GGC-TCG-TGA-TGG-TCA-AG-3′ and antisense: 5-AGG-TCC-ACA-GTA-TTC-TCC-AGG-3′; IRF5: sense: 5′-GGG-CTT-CAA-TGG-GTC-AAC-G-3′ and antisense: 5′-GCC-TTC-GGT-GTA-TTT-CCC-TG-3′. B2M was used as a reference gene, for which the primers were: 5′-ATG-AGT-ATG-CCT-GCC-GTG-TG-3′ (forward) and 5′-CCA-AAT-GCG-GCA-TCT-TCA-AAC-3′ (reverse). The PCR conditions were as follows: 2 min at 50 °C and 10 min at 95 °C, followed by 40 cycles of PCR reaction at 95 °C for 15 s, and 60 °C for 1 min. RNA sequencing RNA sequencing experiments were performed on 4 h unstimulated and C. albicans -stimulated PBMC from three healthy controls and two CMC patients. Total RNA was isolated as described above. The RNA integrity (RNA integrity score ≥7) was measured on the Agilent 2100 Bioanalyzer (Agilent, Santa Clara, USA) using an Agilent RNA 6000 Pico Chip according to the manufacturer's instructions. Enrichment of mRNA was done using the MicroPoly(A)Purist Kit (Ambion, Life Technologies, Foster City, USA) according to manufacturer’s instructions, starting with 5 μg of total RNA and using two rounds of Oligo(dT) selection. Whole transcriptome library preparation was performed using the SOLiD Total RNA-Seq Kit (STaR Kit, Life Technologies) and the corresponding low input amount protocol (version July 2011, Life Technologies). In brief, 25 ng high-quality poly(A) RNA was fragmented by RNAse III digestion, cleaned up using the PureLink RNA Micro Kit (Invitrogen, Life Technologies) and checked for quantity and size-distribution on a Agilent 2100 Bioanalyzer. RNA adapters were hybridized and ligated to the fragmented RNA, followed by reverse transcription. After purification and size-selection of cDNA using Agencourt AMPure XP Reagent beads, the cDNA was amplified and used as input for the SOLiD system bead preparation using the SOLiD Easy bead system (E120 scale). Paired-end sequencing (50+25 bases) was performed on one flowcell of a 5500XL sequencer (Life Technologies) For each sample deep sequencing was performed resulting in a sequencing depth ranging from 75.6 to 105.5 million paired-end reads. Paired-end colorspace reads were mapped against the human genome (hg19) using Tophat (version 1.4.1) [47] . To increase mapping performance a gene transfer format (GTF) file containing the exon boundries of all known RefSeq genes (25,024 genes) was supplied to Tophat and the insert size was set to 110 bases. For all genes FPKM values were calculated using Cufflinks (version 2.0.0) [48] . Further statistical analyses was done using Partek Genomic Suite software (version 6.6, build 6.12.0109, Partek Inc., St Louis, USA). Fold changes and P -values were calculated for each gene by performing a multifactorial ANOVA on log2 (with an offset of 1.0) transformed FPKM expression values. Factors included in the ANOVA model were group (patient or control), treatment (stimulation status), individual (data from same individual) and the interaction between group and treatment. Fold changes for the heatmaps were calculated for each individual by dividing the FPKM expression values of the C. albicans -stimulated sample by the unstimulated (RPMI) sample. Fold changes with values <1 were replaced by the negative of the inverse. A gene list containing 101 differentially expressed transcripts known from the expression array was used to select genes for further downstream analysis. Of this list, 10 transcripts were not considered; 7 because another isoform was already used for FPKM calculations and 3 hypothetical proteins without concordant refseq genes. Accession Codes: Transcriptomics data have been deposited in the Gene Expression Omnibus (GEO) database under accession code GSE42606 . RNA sequencing data have been deposited in the GEO database under accession code GSE42630 . How to cite this article: Smeekens, S.P. et al . Functional genomics identifies type I interferon·pathway as central for host defense against Candida albicans . Nat. Commun. 4:1342 doi: 10.1038/ncomms2343 (2012).